Antibody potency relates to the ability to recognize the closed, pre-fusion form of HIV Env HIV’s envelope glycoprotein (Env) is the sole target for neutralizing antibodies. The structures of many broadly neutralizing antibodies (bNAbs) in complex with truncated Env subunits or components have been reported. However, their interaction with the intact Env trimer, and the structural determinants that underlie neutralization resistance in this more native context are less well understood. Here we use hydrogen/deuterium exchange to examine the interactions between a panel of bNAbs and native-like Env trimers (SOSIP.664 trimers). Highly potent bNAbs cause only localized effects at their binding interface, while the binding of less potent antibodies is associated with elaborate changes throughout the trimer. In conjunction with binding kinetics, our results suggest that poorly neutralizing antibodies can only bind when the trimer transiently samples an open state. We propose that the kinetics of such opening motions varies among isolates, with Env from neutralization-sensitive viruses opening more frequently than Env from resistant viruses. Highly potent, broadly neutralizing antibodies (bNAbs) are now being used to guide the design of an effective HIV-1 vaccine [1] , [2] , [3] . One major obstacle in eliciting a protective, broad humoral immune response has been the high antigenic diversity among circulating isolates. The hypervariable loops present on the surface of the envelope glycoprotein (Env) trimer induce antibodies that are highly isolate-specific and generally lack breadth (as defined by the percent of HIV-1 isolates they can neutralize). The more conserved regions of Env are masked within the trimer before its activation, or are shielded by dense glycosylation; both of these factors restrict the generation of broadly active responses [4] , [5] , [6] , [7] . Despite these viral defenses, a subset of HIV-1-infected individuals can, over time, develop potent (as defined by their IC 50 values in neutralization assays) bNAbs that, in some cases, neutralize >90% of circulating strains [2] , [8] . Structural studies have revealed much about the overall architecture of the Env trimer in its closed, pre-fusion form, including the arrangement of the variable loops at the trimer apex ( Fig. 1a ) [9] , [10] , [11] , [12] . In this conformation, the V3 region is sequestered under the V1/V2 loop structure, while elements of the bridging sheet are involved in quaternary contacts below the V1/V2 loops; together, these interdomain interactions lead to the occlusion of the conserved V3 and bridging sheet elements that are components of the co-receptor binding site [13] , [14] , [15] . Binding of the primary receptor, CD4, induces major structural changes within Env, including the dissociation of contacts between V1/V2 and V3 at the trimer apex and the coalescence of the separate elements of the co-receptor binding site [4] , [16] , [17] , [18] , [19] . 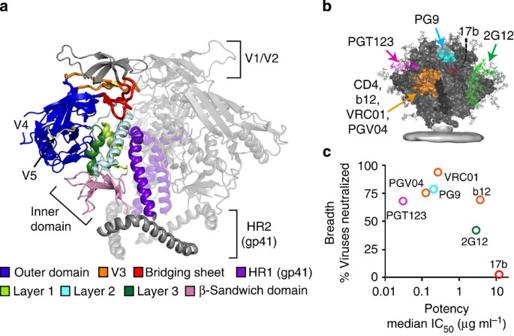Figure 1: Neutralizing antibody targets on Env trimers. (a) The structural elements of gp120 are coloured on one protomer of the closed, pre-fusion Env trimer (PDB accession code: 4NCO)10. (b) The epitopes of the various NAbs used in this study are highlighted on the structure of the closed, pre-fusion trimer. The CD4bs, the target of antibodies b12, VRC01 and PGV04 is shown in orange8,21,22. Glycans at N301 and N332 along the base of V3 make up the PGT123 epitope (magenta)41. The glycan at N160 and nearby residues in V1/V2 constitute the PG9 epitope (cyan)31. Antibody 2G12 recognizes the cluster of glycans at positions N295, N332, N392, N386 and N448 (green)28. Antibody 17b sees the CD4i epitope that is only formed and exposed after CD4 binding23. The viral membrane is shown at the base to illustrate the orientation of Env (electron microscopy databank (EMD) accession code: 5022)9. (c) The breadth (by per cent of viruses neutralized at concentrations <50 μg ml−1) and neutralization potency (median IC50values of the viruses neutralized) are plotted for each NAb. Neutralization data were obtained fromBNAber.org39. Figure 1: Neutralizing antibody targets on Env trimers. ( a ) The structural elements of gp120 are coloured on one protomer of the closed, pre-fusion Env trimer (PDB accession code: 4NCO) [10] . ( b ) The epitopes of the various NAbs used in this study are highlighted on the structure of the closed, pre-fusion trimer. The CD4bs, the target of antibodies b12, VRC01 and PGV04 is shown in orange [8] , [21] , [22] . Glycans at N301 and N332 along the base of V3 make up the PGT123 epitope (magenta) [41] . The glycan at N160 and nearby residues in V1/V2 constitute the PG9 epitope (cyan) [31] . Antibody 2G12 recognizes the cluster of glycans at positions N295, N332, N392, N386 and N448 (green) [28] . Antibody 17b sees the CD4i epitope that is only formed and exposed after CD4 binding [23] . The viral membrane is shown at the base to illustrate the orientation of Env (electron microscopy databank (EMD) accession code: 5022) [9] . ( c ) The breadth (by per cent of viruses neutralized at concentrations <50 μg ml −1 ) and neutralization potency (median IC 50 values of the viruses neutralized) are plotted for each NAb. Neutralization data were obtained from BNAber.org [39] . Full size image Defining how antibodies recognize their epitopes on simple or more complex forms of Env has also shed light on how the trimer functions, and how it resists neutralization ( Fig. 1b ). Antibody b12 was among the first to be generally accepted as broadly neutralizing [20] . Although it recognizes the CD4 binding site (CD4bs), its specific binding footprint is not identical to that of CD4, which restricts its ability to target the native trimer [8] , [21] . More recently identified bNAbs, such as VRC01 (ref. 22 ) and PGV04 (ref. 8 ), more precisely target the CD4bs and have significantly greater breadth and potency. CD4 binding leads to large-scale conformational changes within Env that create a CD4-induced (CD4i) epitope on gp120, the target of some of the earliest known NAbs [23] . One such antibody, 17b, recognizes a portion of the bridging sheet that becomes exposed after CD4 binding; its epitope overlaps with the conserved co-receptor binding site [24] . Although their epitopes are conserved, CD4i antibodies such as 17b generally neutralize only lab-adapted or abnormally sensitive primary viruses (‘tier 1’ isolates) on which the co-receptor binding site is relatively exposed [25] , [26] . Env glycans are also now understood to be wholly or partially involved in the epitopes for several, particularly potent bNAbs. Antibody 2G12 recognizes a conserved patch of high-mannose glycans on the periphery of the CD4bs and has moderate neutralization potency and breadth [27] , [28] , [29] . The more potent PG9/PG16 bNAbs target the V1/V2 structure at the trimer apex via a glycan at N160 (refs 30 , 31 ). Several bNAbs such as PGT123 that interact with the base of V3, including glycans at N301 and N332, are among the most potent yet identified [2] . The different orientations in which many of these antibodies bind various native-like forms of the Env trimer have been described at low to intermediate resolution, via electron microscopy [11] , [17] , [18] , [32] , [33] , [34] . However, critical details of how they bind the trimer and, by extension, neutralize the virus remain to be understood. Although antibody binding is often sufficient to impede the interaction of a trimer with CD4 or the co-receptor, other neutralization mechanisms may involve antibodies locking the trimer in the closed, pre-fusion state or, alternatively, driving its destabilization and inactivation [35] , [36] . Here we use hydrogen/deuterium exchange coupled to mass spectrometry (HDX-MS) to probe the effects of binding of several classes of bNAbs to soluble, native-like Env trimers (SOSIP.664 trimers) [37] . HDX-MS measures the kinetics of deuterium exchange at protein backbone amides. After deuterium exchange under native conditions, the exchange is slowed by acidification (pH 2.5) and low temperature (near 0 °C). The protein is subsequently rapidly digested by an acid-active protease, pepsin, and the resulting peptides are resolved by liquid chromatography–MS to track the kinetics of deuterium exchange throughout the protein. Amides that are engaged in stable hydrogen bonds through secondary structure or that are heavily solvent occluded are protected from exchange, resulting in slow deuterium uptake while amides that are in less structured regions exhibit rapid deuterium uptake [38] . HDX-MS is therefore a sensitive probe of local structural dynamics under native conditions and a particularly powerful tool for monitoring structural changes resulting from ligand binding. We have previously used HDX-MS to probe the solution behaviour of SOSIP.664 trimers and the effects of CD4 binding [19] . Here we now examine the effects of a diverse panel of NAbs against several epitope clusters that span a range of potencies and breadth ( Fig. 1b,c ). The comparisons reveal that the highly potent bNAbs recognize the pre-fusion, closed form of Env, while their less potent counterparts can only recognize more open forms of the trimer. CD4bs-directed antibodies A total of 103 and 120 unique peptides derived from SOSIP.664 trimers could be observed by HDX, resulting in net sequence coverages of 92% and 82% for isolates KNH1144 and BG505, respectively ( Supplementary Figs 1,2 ). To study the interactions of NAbs with the CD4bs, we compared the HDX profiles of unliganded trimers with their complexes with Fabs derived from the highly potent bNAbs VRC01 and PGV04 (IC 50 values of 0.32 and 0.14 μg ml −1 , respectively) and the less potent bNAb b12 (IC 50 , 2.82 μg ml −1 ) [39] . The SOSIP.664 trimers were incubated with a threefold molar excess of each ligand (Fab:monomer) to favour full occupancy ( Supplementary Fig. 3 ). VRC01 exerted only local effects on KNH1144 SOSIP.664 trimers, the changes being limited to increased protection of the CD4 binding loop, V5, Loop D and the α1 helix in layer 2 ( Fig. 2a ). Nearly identical data were obtained for VRC01 and the BG505 SOSIP.664 trimers ( Supplementary Fig. 4a ). All the above changes are localized to regions of gp120 that are in direct contact with the antibody, as judged from the gp120-Fab structure [22] ( Fig. 2c ). Antibody PGV04, which binds the same surface as VRC01 but is even more potent [8] , [11] , caused virtually identical, localized increases in protection ( Supplementary Fig. 4b ). 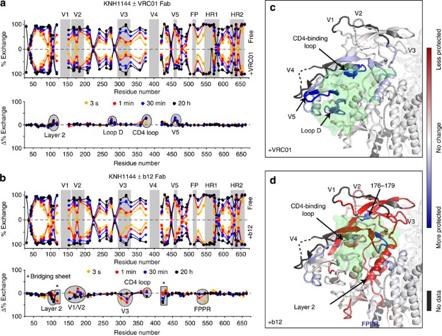Figure 2: Effects of binding of CD4bs-targeting bNAbs. Butterfly plots show the exchange profiles of SOSIP.664 trimers either unliganded (positiveyaxis) or as complexes with (a) VRC01 Fab or (b) b12 Fab (negativeyaxis). The per cent exchange for each observable peptide is plotted at the position of the centre of the peptide on the primary sequence for each time point (3 s to 20 h). The difference plots below each primary plot reveal regions undergoing slower exchange (more protected, above the zero) and faster exchange (less protected, below the zero). Individual plots for the peptides at V1/V2 and V3 are shown inFig. 6, and plots for every peptide are inSupplementary Figs 1 and 2. (c,d) Differences are mapped onto the closed, pre-fusion trimer crystal structure (PDB accession code: 4NCO)10, with regions of faster (red) or slower exchange (blue) in the presence of each antibody highlighted. Segments unresolved in the crystal structure (V2, V4 and FPPR) are shown as dashed lines. As a reference, the binding surfaces of each bNAb on gp120 are shown in green (PDB: 3NGB, 2NY7)21,22. Although b12 binds a more open conformation of the trimer9,17,18, for the sake of comparison all data are illustrated on the closed, pre-fusion structure. Figure 2: Effects of binding of CD4bs-targeting bNAbs. Butterfly plots show the exchange profiles of SOSIP.664 trimers either unliganded (positive y axis) or as complexes with ( a ) VRC01 Fab or ( b ) b12 Fab (negative y axis). The per cent exchange for each observable peptide is plotted at the position of the centre of the peptide on the primary sequence for each time point (3 s to 20 h). The difference plots below each primary plot reveal regions undergoing slower exchange (more protected, above the zero) and faster exchange (less protected, below the zero). Individual plots for the peptides at V1/V2 and V3 are shown in Fig. 6 , and plots for every peptide are in Supplementary Figs 1 and 2 . ( c , d ) Differences are mapped onto the closed, pre-fusion trimer crystal structure (PDB accession code: 4NCO) [10] , with regions of faster (red) or slower exchange (blue) in the presence of each antibody highlighted. Segments unresolved in the crystal structure (V2, V4 and FPPR) are shown as dashed lines. As a reference, the binding surfaces of each bNAb on gp120 are shown in green (PDB: 3NGB, 2NY7) [21] , [22] . Although b12 binds a more open conformation of the trimer [9] , [17] , [18] , for the sake of comparison all data are illustrated on the closed, pre-fusion structure. Full size image As b12 binds poorly to the BG505 SOSIP.664 trimer and fails to neutralize the corresponding virus [40] , only the KNH1144 SOSIP.664 trimer was used to assess what changes resulted from its binding. Unlike with VRC01 and PGV04, changes throughout the trimer were observed with b12 bound. The changes included decreased protection for the majority of V1/V2, V3, layer 2 of the gp120 inner domain and even within the FPPR in gp41, indicating that these regions become more disordered ( Fig. 2b ). Only for the β21 strand of the bridging sheet, residues 176–179 in V2 (sequence FYRL) and the CD4 binding loop (at the early time points) were any increases in protection observed. Based on the b12-Fab structure with core gp120, several of the perturbed regions are not proximal to the binding interface, implying that b12 binding is associated with longer-range structural changes in the trimer ( Fig. 2d ). Glycan-dependent antibodies When the binding of the glycan-dependent antibodies PG9, PGT123 and 2G12 was similarly probed using HDX, we observed only minimal effects on the trimer. As the KNH1144 trimers lack the critical glycan at N160 required for PG9 binding, this complex could only be examined using BG505 trimers. The binding of PG9 resulted in increased protection at only a single site, residues 166–175 in V2 ( Fig. 3a,c ). These residues are known to be proximal to the PG9 epitope, which is centred on the N160 glycan in the crystal structure between PG9 and a V1/V2 scaffold [31] . The mass spectra for the protected peptide in V2 displayed increased peak broadening indicative of the presence of multiple V2 conformations in the PG9-bound trimer (see Supplementary Fig. 5 ). 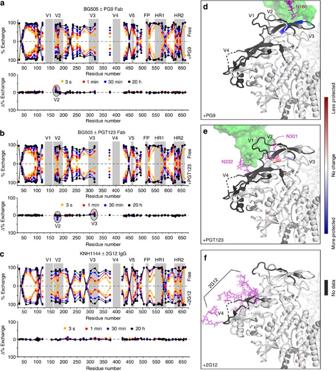Figure 3: Effects of binding of glycan-dependent bNAbs. Butterfly plots show the exchange profiles of SOSIP.664 trimers either unliganded or as complexes with (a) PG9 Fab, (b) PGT123 Fab and (c) 2G12 IgG. The differences are mapped onto the trimer crystal structure (d–f), as described inFig. 2. As a reference, the approximate positions of the Fabs are shown as transparent surfaces (modelled from PDB accession codes 3NGB, 3U4E and 4NCO)70, while glycans known to be relevant to the epitopes are shown as magenta sticks2,28,30. No structure is yet available for the PGT123 trimer complex; hence, PGT122 is shown instead, as its epitope is very similar (PDB: 4NCO)2,10 Figure 3: Effects of binding of glycan-dependent bNAbs. Butterfly plots show the exchange profiles of SOSIP.664 trimers either unliganded or as complexes with ( a ) PG9 Fab, ( b ) PGT123 Fab and ( c ) 2G12 IgG. The differences are mapped onto the trimer crystal structure ( d – f ), as described in Fig. 2 . As a reference, the approximate positions of the Fabs are shown as transparent surfaces (modelled from PDB accession codes 3NGB, 3U4E and 4NCO) [70] , while glycans known to be relevant to the epitopes are shown as magenta sticks [2] , [28] , [30] . No structure is yet available for the PGT123 trimer complex; hence, PGT122 is shown instead, as its epitope is very similar (PDB: 4NCO) [2] , [10] Full size image The binding of the PGT123 Fab to SOSIP.664 trimers also had only minor effects on the HDX profiles. The observed changes were limited to increased protection at the centre of V3 and a small decrease for V2 residues 176–179 ( Fig. 3b ). The affected regions are proximal to the expected PGT123 binding site, as assessed from the electron microscopy and X-ray crystal structures of the complex between the BG505 SOSIP.664 trimer and the closely related bNAb, PGT122 (ref. 41 ) ( Fig. 3d ). Antibody 2G12 has evolved a unique domain swap to enable both Fabs arms to bind to one glycan cluster on gp120 (ref. 42 ). For this reason, 2G12 binding was examined using intact IgG rather than the Fab fragment. The exchange profile showed that 2G12 binding did not change the protection of the underlying protein structure at any site in the trimer ( Fig. 3c,f ), even though the complex was fully formed ( Supplementary Fig. 3a ). Slow binding of the CD4i antibody, 17b Unlike the highly potent bNAbs, the CD4i antibody 17b bound very slowly to the SOSIP.664 trimers. For the KNH1144 trimers, extended incubations of up to 72 h were necessary to generate a homogeneous complex, while no binding of the 17b Fab to their BG505 counterparts could be detected after even this prolonged period ( Fig. 4a,b ). In contrast, soluble two-domain CD4 (sCD4) bound efficiently to both SOSIP.664 trimers within minutes, as did 17b to the CD4-complexed trimers. We note that blue native–polyacrylamide gel electrophoresis (BN–PAGE) gels show only two predominant bands rather than a ladder during the formation of the 17b complex with unliganded KNH1144 SOSIP.664 trimers, suggesting that when binding does occur it is a concerted event involving all three protomers ( Fig. 4b ). 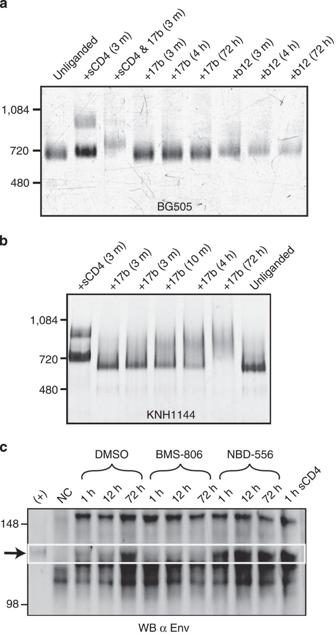Figure 4: Kinetics of 17b Fab binding to SOSIP.664 trimers. (a) BG505 and (b) KNH1144 SOSIP.664 trimers were incubated with ligands for various times (from 3 min to 72 h) and resolved by BN–PAGE. (c) 17b was incubated with KNH1144 SOSIP.664 trimers for various times, the complexes captured by protein G beads, resolved by SDS–PAGE and visualized by immunoblotting. Identical experiments performed in the presence of BMS-806, NBD-556 and sCD4 reveal that NBD-556 and sCD4 both accelerate 17b binding, while BMS-806 blocks it altogether. The gp120 band derived from SOSIP.664 trimers is in the highlighted region marked by the arrow. The other bands represent nonspecific binding of the anti-human serum used as the secondary antibody. Figure 4: Kinetics of 17b Fab binding to SOSIP.664 trimers. ( a ) BG505 and ( b ) KNH1144 SOSIP.664 trimers were incubated with ligands for various times (from 3 min to 72 h) and resolved by BN–PAGE. ( c ) 17b was incubated with KNH1144 SOSIP.664 trimers for various times, the complexes captured by protein G beads, resolved by SDS–PAGE and visualized by immunoblotting. Identical experiments performed in the presence of BMS-806, NBD-556 and sCD4 reveal that NBD-556 and sCD4 both accelerate 17b binding, while BMS-806 blocks it altogether. The gp120 band derived from SOSIP.664 trimers is in the highlighted region marked by the arrow. The other bands represent nonspecific binding of the anti-human serum used as the secondary antibody. Full size image The kinetics of complex formation with 17b were also probed by HDX using a pulse-labelling strategy. Unlike continuous deuterium labelling, here the association time with the ligand is varied, followed by a constant 3-s deuterium pulse. The KNH1144 trimers had bound 17b Fab uniformly after 72 h, while no such binding was detectable for their BG505 counterparts ( Supplementary Fig. 6a,b ). Both BN-PAGE and HDX show that the entire population of KNH1144 SOSIP.664 trimers was present as a 17b complex, and not just a subpopulation. Conversely, the BG505 SOSIP.664 sample contained no subpopulation that was able to bind 17b. SDS–PAGE analysis showed no signs of trimer degradation during the long incubation times used for the experiments above ( Supplementary Figs 3 and 6d ). The rate of 17b binding to unliganded KNH1144 SOSIP.664 trimers was also assessed by immunoprecipitation, which showed that 17b bound slowly, that is, on a timescale of hours to days ( Fig. 4c ). As additional controls, we also tested the rate of 17b binding in the presence of sCD4 and NBD-556 (which both induce the formation of the 17b epitope), and BMS-806 (which inhibits 17b binding) [19] , [43] . In the presence of NBD-556 or sCD4, 17b bound efficiently within 1 h, whereas with BMS-806 there was no 17b binding even after 72 h. In light of the slow binding of 17b, we wondered whether the CD4bs antibody b12 could react better with BG505 trimers if the incubation period was extended. As noted above, b12 binds poorly to BG505 SOSIP.664 trimers, but interacts readily with BG505 gp120 and non-SOSIP gp140, indicating that all necessary contact residues for b12 are present in the BG505 sequence [40] . BN–PAGE analysis showed some evidence of increased smearing of BG505 SOSIP.664 trimers over time, possibly indicating a low level of b12 complex formation ( Fig. 4a ). Using the same HDX pulse-labelling strategy employed with 17b, a change in the V2 region was visible with extended incubations with b12 ( Supplementary Fig. 6c ). Qualitatively, these results suggest that BG505 SOSIP.664 trimers can bind b12 but do so very slowly. This observation is consistent with the lack of neutralizing activity seen with assays that involve a short (30–60 min) incubation period between b12 and the BG505 virus [37] . CD4i antibody binding to SOSIP.664 trimers probed by HDX The HDX profile of the fully formed complex between 17b and the KNH1144 SOSIP.664 trimers showed that extensive changes had occurred throughout the Env protein ( Fig. 5a,c ). Of note is that most of the changes are similar to those seen on sCD4 binding ( Fig. 6a and Supplementary Fig. 4c ), including increased protection throughout portions of the gp120 inner domain and HR1, and the loss in protection for V1/V2, V3 and the FPPR. However, unlike with sCD4, all four strands of the bridging sheet became more protected with 17b binding and no significant change was seen in V5. 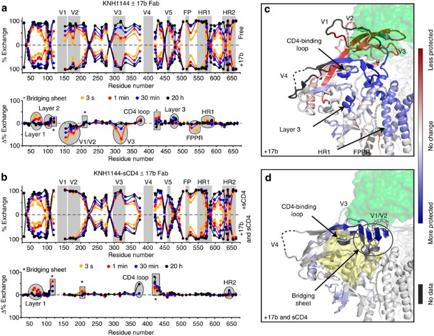Figure 5: Effects of CD4i antibody binding. The butterfly and difference plots compare unliganded SOSIP.664 trimers (isolate KNH1144) with (a) the binary complex with 17b Fab and (b) the ternary complex with sCD4 and 17b Fab. (c) The differences are mapped onto the BG505 SOSIP.664 trimer crystal structure (PDB accession code: 4NCO), as described inFig. 2. Contacts with CD4 (yellow) and Fabs (green) are shown as transparent surfaces (modelled relative to the gp120 core from PDB: 1GC1)24. The regions unresolved in the trimer structure are shown as dashed lines. (d) The effects of 17b binding to sCD4-bound SOSIP.664 trimers are similarly mapped onto the CD4-bound conformation of gp120, as modelled into the trimer structure (PDB: 3JWD)70. The change within HR2 in the ternary complex is not shown, as this region is not resolved in the 4NCO trimer structure. Figure 5: Effects of CD4i antibody binding. The butterfly and difference plots compare unliganded SOSIP.664 trimers (isolate KNH1144) with ( a ) the binary complex with 17b Fab and ( b ) the ternary complex with sCD4 and 17b Fab. ( c ) The differences are mapped onto the BG505 SOSIP.664 trimer crystal structure (PDB accession code: 4NCO), as described in Fig. 2 . Contacts with CD4 (yellow) and Fabs (green) are shown as transparent surfaces (modelled relative to the gp120 core from PDB: 1GC1) [24] . The regions unresolved in the trimer structure are shown as dashed lines. ( d ) The effects of 17b binding to sCD4-bound SOSIP.664 trimers are similarly mapped onto the CD4-bound conformation of gp120, as modelled into the trimer structure (PDB: 3JWD) [70] . The change within HR2 in the ternary complex is not shown, as this region is not resolved in the 4NCO trimer structure. 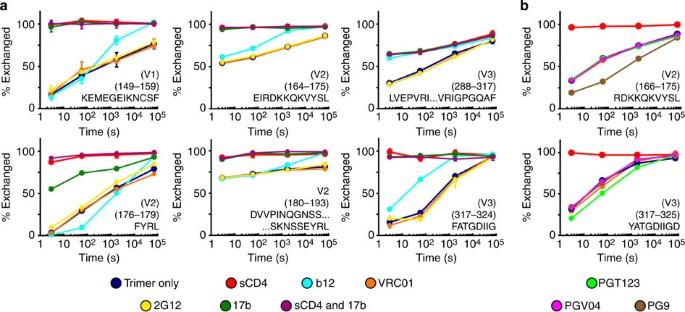Figure 6: Individual exchange profiles of peptides covering V1/V2 and V3. The plots for selected peptides derived from (a) KNH1144 and (b) BG505 SOSIP.664 trimers in unliganded trimer or in complex with sCD4 or various antibodies, as stated. Dots show the mean uptake values at each time point with error bars showing the s.d. between duplicate measurements (in many cases, the error bars are too small to see). Plots for all observable peptides are shown inSupplementary Figs 1 and 2. Full size image Figure 6: Individual exchange profiles of peptides covering V1/V2 and V3. The plots for selected peptides derived from ( a ) KNH1144 and ( b ) BG505 SOSIP.664 trimers in unliganded trimer or in complex with sCD4 or various antibodies, as stated. Dots show the mean uptake values at each time point with error bars showing the s.d. between duplicate measurements (in many cases, the error bars are too small to see). Plots for all observable peptides are shown in Supplementary Figs 1 and 2 . Full size image The sCD4 complex and the ternary complex with sCD4 and 17b were compared, to assess the changes imparted by 17b to the CD4-bound conformation of the KNH1144 SOSIP.664 trimer. The addition of 17b had predominantly local effects near its binding site, with the four strands of the bridging sheet, each becoming substantially more protected ( Fig. 5b,d ). A slight increase in protection was also evident throughout layer 1 of the inner domain and the CD4 binding loop was somewhat more protected within the ternary complex than with sCD4 alone. Finally, there was a small, but reproducible increase in protection for residues 642–645 of gp41 HR2. The collective comparison of the HDX profiles of SOSIP.664 trimers in complex with different classes of bNAbs reveals the extent of allosteric effects imparted by each interaction. With the most potent neutralizing antibodies studied here, the changes on bNAb binding are limited to increased protection at the immediate contact regions ( Figs 2 and 3 ). The highly potent CD4bs antibodies, VRC01 and PGV04, and all the glycan-dependent antibodies had only limited, focused effects on the HDX profiles of the trimers. The glycan cluster-targeting 2G12 antibody had no effects at all on the underlying protein backbone, implying that this epitope does indeed involve only glycans. It remains possible that V4, which is proximal to the 2G12 epitope, undergoes some changes, but this loop could not be monitored by HDX due to its heavy glycosylation. Similarly, PG9 and PGT123 binding may affect more areas of V1/V2 and V3, but as we could not observe peptides that included residues 129–164 and 326–369 we could not monitor changes in those regions ( Supplementary Fig. 2 ). Despite this limitation, the comparisons definitively show that the glycan-dependent antibodies do not exert long-range effects on the protein framework of SOSIP.664 trimers. One peculiarity of PG9 is that it binds asymmetrically to Env trimers with a stoichiometry of 1:1 (Fab:trimer) [32] . Such asymmetric binding would result in complex exchange kinetics, as the three lobes of the trimer would not be affected equally. We observed a subtle broadening in the mass spectrum specifically at V2 within the PG9-bound SOSIP.664 trimer, consistent with the existence of two V2 conformational subpopulations. No such effect was seen with unliganded trimers or any other NAb complex. Qualitatively, the degree of protection indicates that a large proportion of the V2 subdomains become more protected in the PG9 trimer complex. The stabilizing effect of a single bound PG9 Fab therefore probably extends beyond a single lobe of the trimer, which is consistent with our earlier proposal that the binding interface involves two protomers of the trimer [32] . The less potent CD4bs bNAb b12 had a unique effect in that it resulted in changes throughout the KNH1144 SOSIP.664 trimer, with a loss of protection within some of the contact surface ( Fig. 2d ). This outcome is in direct contrast to the purely local effects that were observed with the much more potent CD4bs bNAbs VRC01 and PGV04. Such an unexpected effect probably results from b12 binding to and stabilizing a trimer conformation that has less ordered secondary structure, resulting in faster amide exchange kinetics despite the decreased solvent accessibility arising from solvent occlusion from the protein–protein interface. The binding of b12 also yielded a subtle increase in protection for residues 176–179 within V2 (sequence FYRL), something that was not observed with any of the other antibodies ( Fig. 6 ). A structural alignment to the b12 Fab-gp120 core crystal structure indicated that a portion of the b12 paratope on the trimer is adjacent to this region of V2 ( Fig. 2d ). Hence, residues 176–179, a region absent from the construct used to generate the b12-gp120 core crystal structure, may contribute directly to the b12 epitope. This notion is supported by the substantial effects that mutations involving residues 176–180 have on both b12 binding and neutralization [7] , [44] , [45] . It is noteworthy that 17b can bind to KNH1144 SOSIP.664 trimers, but not their BG505 counterparts, in the absence of CD4. The CD4i epitope is not accessible on the unliganded pre-fusion BG505 SOSIP.664 trimers [10] , [11] . How, then, can 17b bind to the corresponding KNH1144 trimers, albeit with very slow kinetics? As 17b binding in the presence of sCD4 or NBD-556 occurs rapidly, the observed slow binding to the closed trimers (that is, no CD4) cannot simply be explained by a slow intrinsic on-rate ( k on ). We propose that Env trimers, even in the absence of CD4, undergo transient structural fluctuations to sample an open state, and in doing so the CD4i epitope is formed and exposed. This hypothesis would explain the slow binding kinetics of 17b to the unliganded KNH1144 SOSIP.664 trimers; specifically, 17b binds only to the transiently open state of the trimers, forming a complex primarily via conformational selection ( Fig. 7a ). This concept is also consistent with the coordinated binding of three 17b Fabs per trimer (that is, the lack of evidence for partial occupancy). Thus, once opened, the binding of 17b to a single lobe of the trimer blocks the re-formation of the quaternary interactions at the apex, which means that the other two lobes remain accessible for the rapid binding of two more 17b Fabs. In contrast to 17b, CD4 binds rapidly to the trimer, suggesting that major conformational transitions do not need to occur before binding. Instead, it is the CD4 binding event itself that most probably leads to large-scale conformational changes in the trimer ( Figs 4 and 7a ). 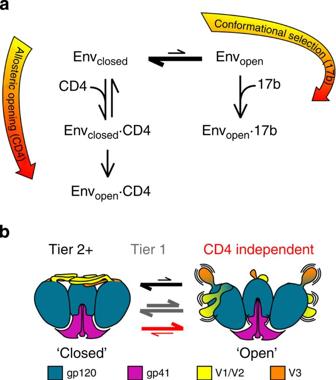Figure 7: Conformational sampling of unliganded Env trimers. (a) CD4 can bind the closed form of Env and allosterically induce an open conformation. In contrast, 17b can only bind to unliganded Env when the open conformation is transiently sampled, and by doing so it stabilizes this conformation. (b) Env trimers exist predominantly in the closed form in which the interactions between V1/V2 from each protomer are intact and V3 is occluded. Transient sampling of open conformations disrupts the inter-protomer interactions at the trimer apex. The trimers on higher tier (more neutralization-resistant) viruses are less likely to sample open conformations, thereby protecting conserved epitopes from NAbs. Tier 1 primary and cell line-adapted isolates sample the open conformation more often or for longer periods, which renders these viruses more vulnerable to neutralization. CD4-independent isolates (which are extremely neutralization sensitive) have evolved mutations that stabilize the open state, probably to facilitate co-receptor binding when CD4 is either present at low levels or entirely absent. Figure 7: Conformational sampling of unliganded Env trimers. ( a ) CD4 can bind the closed form of Env and allosterically induce an open conformation. In contrast, 17b can only bind to unliganded Env when the open conformation is transiently sampled, and by doing so it stabilizes this conformation. ( b ) Env trimers exist predominantly in the closed form in which the interactions between V1/V2 from each protomer are intact and V3 is occluded. Transient sampling of open conformations disrupts the inter-protomer interactions at the trimer apex. The trimers on higher tier (more neutralization-resistant) viruses are less likely to sample open conformations, thereby protecting conserved epitopes from NAbs. Tier 1 primary and cell line-adapted isolates sample the open conformation more often or for longer periods, which renders these viruses more vulnerable to neutralization. CD4-independent isolates (which are extremely neutralization sensitive) have evolved mutations that stabilize the open state, probably to facilitate co-receptor binding when CD4 is either present at low levels or entirely absent. Full size image The argument that 17b recognizes an open form of Env trimers is further supported by the HDX comparisons. All the major changes associated with the opening of the trimer, including loss of protection at V1/V2 and V3, were observed in the 17b complex ( Fig. 6 ). There were only two major differences between the 17b- and sCD4-bound data sets: (1) for 17b, there was increased protection throughout the bridging sheet, which is in direct contact with the Fab and (2) for sCD4, there was more protection at V5, which is involved in the binding interface for sCD4 but not 17b. When 17b binds to the already opened sCD4-SOSIP.664 trimer complex, the major changes involve stabilization of the regions in direct contact with the Fab ( Fig. 5d ). We noted that the binding of b12 also caused changes throughout the trimer, with portions of V1/V2 and V3 losing protection. Together with the slow binding of b12 Fab to the BG505 SOSIP.664 trimers, this finding suggests that similar to 17b, b12 recognizes an open conformation of the trimer. The current study demonstrates that highly potent bNAbs target the closed conformation of Env without inducing conformational changes, something that has been observed for several other Ab–pathogen systems [35] . Less-potent antibodies (for example, b12) may require the trimer to transiently sample partially open states in which their epitopes are exposed. Antibodies such as 17b whose epitopes are masked in the closed trimer conformation are likely to recognize only the fully open trimer conformation in which the co-receptor binding site is unmasked and its elements assembled. This trend is consistent with low resolution cryo-electron tomography studies, which reported that sCD4 and 17b binding resulted in open trimer conformations, that b12 binding caused the trimer to partially open, and that VRC01 binding caused no such opening [9] , [17] , [18] . Furthermore, both CD4 and b12 have been observed to induce gp120 shedding from virus, a presumed marker of substantial conformational changes, whereas VRC01 and PGV04 do not have such an effect [45] , [46] . It is relevant to draw a distinction between what happens when NAbs bind to the gp120 subunits of trimers compared with individual gp120 monomers. For example, VRC01 binding to gp120 monomers is associated with a large entropic penalty, suggesting that gp120 transitions from a highly dynamic form to a more constrained conformation [45] . In contrast, b12 binding to monomeric gp120 is associated with a much less significant change in entropy, suggestive of a less profound structural change [5] . This pattern is the inverse of what we see when the same two NAbs interact with the trimer; the probable explanation is that gp120 in the trimer context is more conformationally constrained then when it is an isolated monomer, particularly with respect to V1/V2, V3 and the bridging sheet [10] , [11] , [12] , [19] , [47] . Moreover, quaternary steric hindrance effects restrict how b12 can gain access to the CD4 binding site on the closed, pre-fusion trimer [9] , [17] , a constraint that is absent from monomeric gp120. The highly ordered, unliganded conformation of the Env trimer in which the trimer apex is formed by the V1/V2 and V3 loops, and in which conserved epitopes such as the co-receptor binding site are masked, is often referred to as the ‘closed’ conformation or ‘ground state’ [48] . The binding of CD4 induces profound allosteric changes such that the trimer adopts an ‘open’ configuration, with the quaternary associations between V1/V2 and V3 at the trimer apex now released. Cryo-electron tomography images of the unliganded (closed) and CD4-bound (fully open) trimer provide a low-resolution, but highly informative, view of these two states [9] , [17] , [18] . We note that a much earlier usage of the ‘open/closed’ terminology refers to the conformations of Env on viruses, as inferred from their neutralization phenotypes. In the 1990s, it was common to refer to neutralization-sensitive (usually cell line adapted) viruses as having a more open (that is, antibody accessible) form of Env than their resistant, primary isolate counterparts [49] , [50] , [51] , [52] . The phenotypic difference between the neutralization-sensitive, cell line-adapted, tier 1 isolates and more resistant primary isolates (now categorized as tier 2 or 3) has been attributed to undefined aspects of the quaternary structure of their trimers [7] , [26] , [53] , [54] . A very recent paper emphasizes the critical role of the V2 loop in these neutralization phenotypes, probably via influences on the formation and stability of the inter-protomer associations at the trimer apex [55] . Here we propose that the subtly differing open/closed terminologies may be manifestations of a single phenomenon: the transient opening motions of the trimer that occur at different rates among different isolates that are a major determinant of neutralization susceptibility ( Fig. 7b ). Under the immune pressures that target conserved regions such as the co-receptor binding site, the more neutralization-resistant isolates have evolved Env trimers that better mask conserved epitopes by sampling the open conformations only transiently and infrequently [48] , [49] , [50] , [56] , [57] . Conversely, cell line-adapted isolates that were cultured in the absence of antibody selection pressures evolved to sample the open state more readily. CD4-independent isolates, which can enter cells that lack CD4 but express the co-receptor, are extremely susceptible to neutralization [58] , [59] and primarily exist in the open state [16] . This trend is consistent with the recent observation that a higher level of ‘intrinsic reactivity’ (ability of Env to sample different conformations) correlates with sensitivity to antibody neutralization [60] . Our study is limited to the KNH1144 and BG505 SOSIP.664 constructs, which represent the only soluble native-like Env trimers currently available. Examination of native-like trimers from other isolates will be necessary for a complete understanding of the relationship between the kinetics of Env’s transient opening motions and neutralization susceptibility. Although our HDX analysis has revealed much about the conformational state of the trimer, under the current conditions it does not appear to provide a quantitative measure of the kinetics of transient opening motions. If the open conformations persisted in solution on a long timescale (seconds), then it would result in correlated exchange kinetics (EX1 regime) as evidenced by bimodal mass spectra under our experimental conditions [61] . However, no such EX1 behaviour was observed for the unliganded trimer and all portions of the protein exchange through fast local structural fluctuations (EX2). Furthermore, ligands that are expected to stabilize the closed conformation (for example, PG9) only show local effects at their binding site, without altering the HDX profile through the rest of the trimer apex. Likewise, under the experimental conditions used, SOSIP.664 from BG505 and KNH1144 isolates had very similar HDX profiles, despite phenotypic differences. For one, KNH1144 has lower thermal stability than BG505 trimers [19] , [32] . The kinetics of b12 and 17b binding are also drastically different between the two isolates, indicating a lower frequency of exposure of several epitopes in BG505. The relative kinetics of ligand binding to the partially open (with b12) or fully open (with 17b) form of the trimer should serve as an additional assay for assessing the degree of transient opening motions within different Env trimers. Recently, single-molecule fluorescence experiments have demonstrated that native Env on the membrane samples transient open states, and that potent neutralizing antibodies stabilize the closed state of the trimer [12] , [48] . Furthermore, in agreement with our own observations, the transient fluctuations to the activated (open) states were more frequent with neutralization-sensitive isolates. Despite any caveats that may be associated with the use of soluble SOSIP.664 trimers (that is, the presence of stabilizing mutations and the absence of the MPER/transmembrane segments of gp41), their properties and behaviour do appear to reflect what is observed using full-length, fusion-competent Env trimers. Beyond the concurrence in behaviours between soluble SOSIP.664 trimers and Env on virus, characterizing the interaction of the SOSIP trimer with antibodies provides valuable information for understanding its properties as a potential immunogen. The development of broadly cross-reactive antibodies is relatively uncommon during the course of HIV-1 infection and generally takes several years when it does happen [62] . In light of the fact that all of the highly potent bNAbs target the closed form of Env, more potent Ab responses may be achieved by using trimer immunogens that present the closed form of Env as stably as possible. For such immunogens, any transient sampling of open conformations should be minimized to avoid exposing undesirable, non-neutralizing epitopes that could potentially distract the humoral immune response. The BG505 SOSIP.664 protein appears to embody such an immunogen that presents the major neutralizing epitopes in the context of a stable, closed trimer [37] . The contrast between the KNH1144 and BG505 SOSIP.664 trimers, which bind 17b slowly versus not at all, implies that the BG505 trimers are the more likely to remain in the fully closed state, sampling the open state(s) less frequently than their KNH1144 counterparts. Further modifications to the BG505 SOSIP.664 trimers may be useful for reducing the spontaneous or CD4-induced opening of the trimer that is likely to occur in vivo during the course of vaccination. Identifying other closed conformation, native-like trimers with comparable properties is an additional priority, not least to allow the exploration of more complex immunization regimens. Sample preparation SOSIP.664 trimers based on the subtype A isolates KNH1144 and BG505 were expressed in 293S GnTI−/− cells and purified by 2G12 affinity followed by size-exclusion chromatography (Superdex S200, GE Healthcare) in PBS (20 mM sodium phosphate pH 7.4, 150 mM NaCl with 1 mM EDTA and 0.02% sodium azide) as described previously [19] , [63] . sCD4 (ref. 64 ), HIV-IG and monoclonal antibodies 17b [4] , [14] , [23] , [24] , b12 (refs 20 , 65 , 66 ), 2G12 (refs 27 , 67 ) and VRC01 (ref. 68 ) were obtained from the NIH AIDS reagents programme. Fabs were prepared using Pierce Fab preparation kit (Thermo Scientific) according to manufacturer’s instructions. PGV04, PGT123 and PG9 Fabs were prepared as described previously [69] . All proteins were buffer exchanged into PBS. Complexes with SOSIP.664 trimers were formed by overnight incubation with a threefold molar excess of ligand (relative to each protomer) at 4 °C, except for the 17b Fab complex, which was incubated for 72 h at room temperature. SDS– and BN–PAGE analyses were performed with the same samples used for HDX, to ensure that complexes had formed and that no degradation had occurred throughout the incubations ( Supplementary Fig. 3 ). Hydrogen/deuterium exchange SOSIP.664–antibody complexes (15 μg) were diluted tenfold into deuterated PBS buffer and incubated at room temperature. Aliquots removed after 3 s, 1 min, 30 min and 20 h were quenched by mixing with an equal volume of cold 200 mM Tris-2-carboxyethyl phosphine, 0.2% formic acid (final pH 2.5). The samples were subsequently digested with pepsin (at 0.15 mg ml −1 ) for 5 min on ice, flash frozen in liquid nitrogen and stored at −80 °C. For liquid chromatography–MS analysis, samples were thawed on ice for 5 min and manually injected onto a Waters BEH 1.7 μm, 1.2 × 5 mm trap column (Waters) flowing 0.1% TFA at 200 μl min −1 . After 3 min of washing, the peptides were resolved over a Hypersil 1 × 50 mm, 2.1 μm C18 column (Thermo Scientific), using a gradient of 15%–40% B in 8 min (A: 0.05% TFA, 5% ACN; B: 0.05% TFA, 80% ACN). Two hundred microlitres of 10% formic acid, 80% MeOH, 2:1 IPA:ACN and 80% ACN were injected over the loop and trap column between injections, while two rapid (10%–100% B in 30 s) gradients were used to clean the resolving column, to minimize carryover. Eluting peptides were analysed with a Waters Synapt Q-TOF mass spectrometer, with source and desolvation temperatures of 80°C and 150 °C, respectively. Peptic peptides were identified by exact mass and MS/MS spectra. Identification of glycopeptides was aided by MS/MS spectra of the fully deglycosylated samples as described previously [19] . Per cent exchange for each time point was calculated relative to zero and fully deuterated standards as described previously [47] . For ligand binding kinetics, SOSIP.664 trimers at 1 mg ml −1 were incubated with a threefold excess of b12 or 17b Fab in PBS at 22 °C. At 3 min, 4 h and 72 h, an aliquot of the mixture was diluted tenfold into deuterated PBS buffer for 3 s and rapidly quenched. Antibody binding assays The kinetics of 17b binding were measured by incubating SOSIP.664 trimers at 1 mg ml −1 with a threefold molar excess of 17b Fab (relative to protomers) and a monitoring complex formation by BN–PAGE. Immunoprecipitation experiments were initiated by addition of 2 μg of 17b Fab to 3 μg of KNH1144 SOSIP.664 trimers in 120 μl of PBS plus 2% dimethyl sulfoxide, together with the following: no ligand, 100 μM NBD-556, 100 μM BMS-806 or 0.4 μM of sCD4. Pre-washed protein G sepharose beads were added after the mixtures were incubated at 25 °C for various times, and rotated on a nutator for 1 h. The beads were pelleted by centrifugation and washed four times in PBS plus 0.1% Tween 20, followed by re-suspension and boiling in reducing SDS-gel loading buffer (Invitrogen). Western blottings were probed with HIV-Ig serum (1:1,000 dilution), followed by anti-human-horseradish peroxidase (1:5,000 dilution; Jackson Immunoresearch). The labelled bands were visualized by chemilluminescence (Western lightning, Perkin Elmer). How to cite this article: Guttman, M. et al. Antibody potency relates to the ability to recognize the closed, pre-fusion form of HIV Env. Nat. Commun. 6:6144 doi: 10.1038/ncomms7144 (2015).